Gipc3mutations associated with audiogenic seizures and sensorineural hearing loss in mouse and human Sensorineural hearing loss affects the quality of life and communication of millions of people, but the underlying molecular mechanisms remain elusive. Here, we identify mutations in Gipc3 underlying progressive sensorineural hearing loss (age-related hearing loss 5, ahl5 ) and audiogenic seizures (juvenile audiogenic monogenic seizure 1, jams1 ) in mice and autosomal recessive deafness DFNB15 and DFNB95 in humans. Gipc3 localizes to inner ear sensory hair cells and spiral ganglion. A missense mutation in the PDZ domain has an attenuating effect on mechanotransduction and the acquisition of mature inner hair cell potassium currents. Magnitude and temporal progression of wave I amplitude of afferent neurons correlate with susceptibility and resistance to audiogenic seizures. The Gipc3 343A allele disrupts the structure of the stereocilia bundle and affects long-term function of auditory hair cells and spiral ganglion neurons. Our study suggests a pivotal role of Gipc3 in acoustic signal acquisition and propagation in cochlear hair cells. Degeneration of the sensory hair cells in the organ of Corti and their innervating afferent neurons in the cochlear spiral ganglion results in sensorineural hearing loss (SNHL), which typically begins at the higher frequencies (>15 kHz) and gradually affects lower frequencies. SNHL is among the most common sensory impairment affecting ∼ 17% of adult Americans. Age-related hearing impairment (ARHI) or presbycusis impairs 30% of adults older than 65 years in the US [1] . Heritability and twin studies have suggested genetic contributions to presbycusis and a genome-wide-association study recently identified a genetic variant in the metabotropic glutamate receptor 7 ( GRM7 ) gene as a risk factor [2] , [3] , [4] , [5] . However, the majority of the genetic variation underlying susceptibility to SNHL remains unknown. Progressive SNHL in mice displays a histopathology similar to that in humans [6] , [7] , [8] , [9] . Extensive natural variation in mouse strains has caused a remarkable phenotypic and genetic heterogeneity of SNHL, providing experimental model systems to systematically decipher the underlying risk factors [10] . We recently identified an early-onset hearing loss in Black Swiss (BLSW) mice that is controlled by the quantitative trait loci (QTL) age-related hearing loss 5 ( ahl5 ) and ahl6 (ref. 11 ), whereby the ahl5 QTL accounts for ∼ 60% of the variation observed. The 95% confidence interval for ahl5 is localized to a 25 Mbp region on chromosome 10 ( D10Mit20 - D10Mit95; 66, 475–91, 965 kbp). BLSW mice are also sensitive to acoustic stimulation, responding to loud noise with seizures, characterized by wild running, and tonic and clonic convulsions [12] . Sensitivity to audiogenic seizures is highest at 2–3 weeks of age, but then susceptibility gradually decreases and mice become resistant at 6 weeks of age. The underlying locus, juvenile audiogenic monogenic seizure 1 ( jams1 ), localizes to a 1.6cM region that overlaps with the ahl5 interval [12] . The genetic location and their related pathology suggested that the ahl5 and jams1 phenotypes are caused by the same allele as previously shown for the 6748delG mutation in the Gpr98 gene causing both audiogenic seizures and hearing loss in the Frings and BUB/BnJ mouse strains [13] , [14] . The Gipc (GAIP interacting protein, C terminus) genes encode a small family of proteins characterized by a single, centrally located PDZ domain [15] . GIPC1 was first identified through its interaction with regulator of G-protein signalling 19 ( Rgs19 ) and has now been shown to interact with a host of proteins that are involved in signal transduction, vesicular trafficking, endocytosis and neurotransmitter release [16] , [17] , [18] , [19] , [20] . Using its carboxy (C) terminal domain, GIPC1 was demonstrated to interact with Myosin VI, which is associated with SNHL in both mice and humans [21] , [22] , [23] . Loss of Gipc1 function ( Gipc1 tm1Mvc ) results in a reduction in pre- and postsynaptic transmission in hippocampal neurons [19] . Here, we identified a sequence polymorphism in the PDZ domain of Gipc3 as the cause of SNHL ( ahl5 ) and audiogenic seizure susceptibility ( jams1 ) in BLSW mice and we implicate mutations in GIPC3 in human recessive SNHL (DFNB15 and DFNB95). Our study suggests a critical role of Gipc3 in signal acquisition and propagation in auditory hair cells. Positional cloning of ahl5 To genetically refine the ahl5 region, we generated two congenic lines, 10.R and 10.2, by serial backcrossing normal hearing BLSW.CAST- +/ahl5 progeny to BLSW mice. At generation N8 and higher, there was a significant correlation between segregation of ahl5 alleles and auditory brain stem response (ABR) thresholds ( Fig. 1a ). Recombination events delimited the ahl5 interval to a 2.19 Mbp region ( Fig. 1b and Supplementary Fig. S1 ). We sequenced 735 of the 831 coding exons in BLSW genomic DNA and identified one nucleotide substitution, which was a guanine to adenine transition in exon 2 of the Gipc3 gene (c.343G>A; Fig. 1c,d ). The mutation was absent in 14 inbred and four heterogeneous mouse strains (NMRI, Swiss Webster, CF1 and ICR). However, the 343G/A alleles segregated in mice of the National Institutes of Health (NIH) Swiss founder strain and showed significant correlation with hearing status. Gipc3 343A/A homozygotes had impaired hearing (95±7 dBSPL at 16 kHz), whereas NIH Swiss mice homozygous at the wild-type allele ( Gipc3 343G/G ) exhibited normal hearing (16±5 dBSPL at 16 kHz; Fig. 1e ). The missense mutation replaced a glycine with an arginine at position 115 (Gly115Arg) located within the PDZ domain (aa107–174). The Gly115 residue is highly conserved, showing 100% identity in all published GIPC protein sequences in animals and plants ( Fig. 1f ). 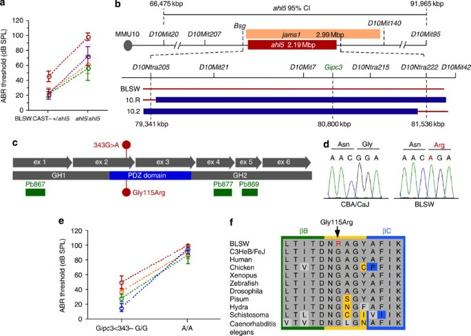Figure 1: Positional cloning of theahl5locus. (a) ABR thresholds at click (orange), 8 (green), 16 (purple) and 32 kHz (red) of congenic BLSW.CAST-+/ahl5 (n=83) and BLSW.CAST-ahl5/ahl5(n=59) mice at 8 weeks of age. Hearing thresholds (dBSPL) were significantly elevated for the BLSW.CAST-ahl5/ahl5animals compared with BLSW.CAST-+/ahl5(ANOVA,P<0.001). Data are given as mean±s.d. (b) Theahl595% confidence interval (CI) on chromosome 10 (MMU10) defined by markersD10Mit20andD10Mit95is shown. Refined genotyping of two congenic lines 10.R and 10.2 delimited theahl5critical interval in a 2.19 Mbp region (red box) defined by markersD10Ntra205andD10Ntra222. Blue bars at the bottom of the map represent the congenic segments from CAST/EiJ introgressed onto the BLSW genetic background (red lines). Thejams1locus delimited by the gene Basigin (Bsg) and markerD10Mit140on MMU10 is shown (orange box)12. Physical location ofGipc3within theahl5interval is given. Position of the markers is given in kilobase pairs (kbp). (c)Gipc3has six exons and is predicted to encode a 297 amino-acid protein with a central PDZ domain (blue box) flanked by amino- and C-terminal GIPC homologous domains GH1 and GH2 (grey boxes). Position of the mutation (red annotation) and polyclonal antisera Pb867, Pb869 and Pb877 (green boxes) is shown. (d) Sequencing chromatograms demonstrating the 343G>A transition in wild-type (left) and mutant (right) are shown. The nucleotide (A, adenine) and amino acid (Arg, arginine) changes are shown in red. (e) ABR thresholds (dBSPL) at click (orange), 8 (green), 16 (purple) and 32 kHz (red) of NIH Swiss homozygous for the wild-type (343G/G;n=9) and mutant (343A/A;n=9)Gipc3alleles. Homozygous (343A/A) NIH Swiss at 6 weeks of age had significantly higher thresholds at all tested stimuli (P<0.0001; ANOVA). Data are given as mean±s.d. (f) ClustalW alignment of the amino-acid sequence of Gipc3 homologues and the location of the Gly115Arg relative to the secondary structure, obtained from the GIPC2 crystal structure (DOI:10.2210/pdb3gge/pdb) is shown. Gly115 maps to a loop (yellow), connecting to β strands, βB (green) and βC (blue). Figure 1: Positional cloning of the ahl5 locus. ( a ) ABR thresholds at click (orange), 8 (green), 16 (purple) and 32 kHz (red) of congenic BLSW.CAST- +/ahl5 (n =83) and BLSW.CAST- ahl5/ahl5 ( n =59) mice at 8 weeks of age. Hearing thresholds (dBSPL) were significantly elevated for the BLSW.CAST- ahl5/ahl5 animals compared with BLSW.CAST- +/ahl5 (ANOVA, P <0.001). Data are given as mean±s.d. ( b ) The ahl5 95% confidence interval (CI) on chromosome 10 (MMU10) defined by markers D10Mit20 and D10Mit95 is shown. Refined genotyping of two congenic lines 10.R and 10.2 delimited the ahl5 critical interval in a 2.19 Mbp region (red box) defined by markers D10Ntra205 and D10Ntra222 . Blue bars at the bottom of the map represent the congenic segments from CAST/EiJ introgressed onto the BLSW genetic background (red lines). The jams1 locus delimited by the gene Basigin ( Bsg ) and marker D10Mit140 on MMU10 is shown (orange box) [12] . Physical location of Gipc3 within the ahl5 interval is given. Position of the markers is given in kilobase pairs (kbp). ( c ) Gipc3 has six exons and is predicted to encode a 297 amino-acid protein with a central PDZ domain (blue box) flanked by amino- and C-terminal GIPC homologous domains GH1 and GH2 (grey boxes). Position of the mutation (red annotation) and polyclonal antisera Pb867, Pb869 and Pb877 (green boxes) is shown. ( d ) Sequencing chromatograms demonstrating the 343G>A transition in wild-type (left) and mutant (right) are shown. The nucleotide (A, adenine) and amino acid (Arg, arginine) changes are shown in red. ( e ) ABR thresholds (dBSPL) at click (orange), 8 (green), 16 (purple) and 32 kHz (red) of NIH Swiss homozygous for the wild-type (343G/G; n =9) and mutant (343A/A; n =9) Gipc3 alleles. Homozygous (343A/A) NIH Swiss at 6 weeks of age had significantly higher thresholds at all tested stimuli ( P <0.0001; ANOVA). Data are given as mean±s.d. ( f ) ClustalW alignment of the amino-acid sequence of Gipc3 homologues and the location of the Gly115Arg relative to the secondary structure, obtained from the GIPC2 crystal structure (DOI:10.2210/pdb3gge/pdb) is shown. Gly115 maps to a loop (yellow), connecting to β strands, βB (green) and βC (blue). Full size image SNHL and audiogenic seizures in BLSW At 4 weeks of age, BLSW mice showed a moderate hearing impairment with mean thresholds significantly elevated for the click, 8, 16 and 32 kHz stimuli (68±7, 41±6, 41±5 and 85±5 dBSPL) compared with thresholds of 4-week-old normal hearing C3HeB/FeJ mice ( P <0.001). At 52 weeks of age, BLSW mice exhibited a profound hearing loss that progressed from higher to lower test frequencies. The increase in hearing thresholds was most pronounced at 16 kHz with a shift of 48 dBSPL over the threshold of 4-week-old BLSW mice ( Fig. 2a ). 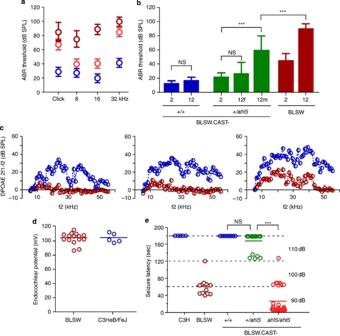Figure 2: Sensorineural hearing loss and audiogenic seizures in BLSW. (a) ABR thresholds (dBSPL) of BLSW at 4 (orange symbol,n=18) and 52 (red,n=20) weeks age compared with 4-week-old C3HeB/FeJ (blue,n=9) are given as mean±s.d. (b) ABR thresholds (dBSPL) at the 16k Hz stimulus in 2- (n=6) and 12-months-old (n=17) BLSW.CAST-+/+ (blue), and in 2-month-old BLSW.CAST-+/ahl5(green,n=52), and 2- (n=9) and 12-months-old (n=20) BLSW (red) are given as mean±s.d. ABR thresholds in 12-month-old females (12f,n=30) and males (12 m,n=30) are given. NSP>0.05, ***P<0.001 (ANOVA). (c) DPOAE levels (dBSPL) at the 2f1-f2 frequency are plotted against the f2 frequency (kHz) for 55 dBSPL (left), 65 dBSPL (middle) and 75 dBSPL (right) L2 levels. Emission levels relative to noise floor of C3HeB/FeJ (blue,n=25) and BLSW (red,n=16) mice at 4 weeks of age are given as mean±s.e.m. (d) Endocochlear potential measurements of C3HeB/FeJ (blue,n=5) and BLSW (red,n=15) mice. Each circle refers to one measurement and the lines indicate the mean in each strain. Values are given in millivolt (mV). (e) Audiogenic seizure susceptibility of C3HeB/FeJ (blue,n=5), BLSW (dark red,n=14) and congenic BLSW.CAST-+/+ (blue,n=9), BLSW.CAST-+/ahl5(green,n=23), BLSW.CAST-ahl5/ahl5(light red,n=34) at 3 weeks of age using white noise stimuli of 90, 100 and 110 dBSPL (dotted lines). Each circle represents one animal and lines indicate the mean of the seizure latency of each strain in seconds. NSP>0.05; ***P<0.001. NS, not significant. Figure 2: Sensorineural hearing loss and audiogenic seizures in BLSW. ( a ) ABR thresholds (dBSPL) of BLSW at 4 (orange symbol, n =18) and 52 (red, n =20) weeks age compared with 4-week-old C3HeB/FeJ (blue, n =9) are given as mean±s.d. ( b ) ABR thresholds (dBSPL) at the 16k Hz stimulus in 2- ( n =6) and 12-months-old ( n =17) BLSW.CAST-+/+ (blue), and in 2-month-old BLSW.CAST- +/ahl5 (green, n =52), and 2- ( n =9) and 12-months-old ( n =20) BLSW (red) are given as mean±s.d. ABR thresholds in 12-month-old females (12f, n =30) and males (12 m, n =30) are given. NS P >0.05, *** P <0.001 (ANOVA). ( c ) DPOAE levels (dBSPL) at the 2f1-f2 frequency are plotted against the f2 frequency (kHz) for 55 dBSPL (left), 65 dBSPL (middle) and 75 dBSPL (right) L2 levels. Emission levels relative to noise floor of C3HeB/FeJ (blue, n =25) and BLSW (red, n =16) mice at 4 weeks of age are given as mean±s.e.m. ( d ) Endocochlear potential measurements of C3HeB/FeJ (blue, n =5) and BLSW (red, n =15) mice. Each circle refers to one measurement and the lines indicate the mean in each strain. Values are given in millivolt (mV). ( e ) Audiogenic seizure susceptibility of C3HeB/FeJ (blue, n =5), BLSW (dark red, n =14) and congenic BLSW.CAST-+/+ (blue, n =9), BLSW.CAST- +/ahl5 (green, n =23), BLSW.CAST- ahl5/ahl5 (light red, n =34) at 3 weeks of age using white noise stimuli of 90, 100 and 110 dBSPL (dotted lines). Each circle represents one animal and lines indicate the mean of the seizure latency of each strain in seconds. NS P >0.05; *** P <0.001. NS, not significant. Full size image The availability of the BLSW.CAST- +/ahl5 congenic lines allowed us to evaluate the effect of ahl5 on the progression of the hearing loss. BLSW.CAST-+/+ mice showed normal hearing at 2 and 12 months of age with mean thresholds of 12±4 and 16±5 dBSPL for the 16 kHz stimulus, respectively ( Fig. 2b ). BLSW.CAST-+ /ahl5 heterozygotes had normal thresholds at 2 months of age (21±6 dBSPL), but exhibited significantly elevated thresholds at 12 months. This increase was more prominent in males (57±23 dBSPL) than in females (25±16 dBSPL; P <0.001, analysis of variance (ANOVA)). The threshold increase in 12-month-old female heterozygotes was modest with large standard deviations, but the difference compared with 2-month-old females was not significant. Last, the elevated thresholds of male heterozygotes were lower than the thresholds in 12-month-old BLSW mice (89±7 dBSPL). These results suggest that a gender– ahl5 interaction controls the progression of hearing loss in BLSW.CAST- +/ahl5 heterozygotes. We next measured distortion product otoacoustic emissions (DPOAEs), which are an indicator of outer hair cell (OHC) function. At 4 weeks of age, DPOAEs were reduced at the 5–20 kHz f2 frequencies (L2=65 dBSPL) and were absent between 20 and 55 kHz compared with normal hearing C3HeB/FeJ mice at the same age ( Fig. 2c ). To test for a defect in the stria vascularis, we measured the endocochlear potential (EP). In 10-week-old BLSW mice, the EP was 104±8 mV, which was comparable with potentials obtained from C3HeB/FeJ mice (105±7 mV; Fig. 2d ). Together, the data suggest that BLSW mice exhibit progressive SNHL. To test whether jams1 localized to the ahl5 critical region, we tested BLSW.CAST congenic mice for audiogenic seizure susceptibility. An acoustic stimulus of 90–100 dBSPL for the duration of 61±20 s readily induced a seizure response in 3-week-old BLSW mice. Age-matched C3HeB/FeJ mice showed no seizing activity after 180 s at 110 dBSPL ( P <0.001). Likewise, BLSW.CAST- ahl5/ahl5 homozygotes were highly susceptible to white noise stimulation showing a rapid seizure response (27±31 s). In contrast, BLSW.CAST-+/+ showed no signs of audiogenic seizures (180 s) exhibiting a response identical to that of C3HeB/FeJ mice (180 s, P >0.05; Fig. 2e ). In addition, although five BLSW.CAST- +/ahl5 responded with convulsions at the highest 110 dBSPL stimulus (132±4 s), most of the BLSW.CAST- +/ahl5 mice were resistant to seizure induction (180 s, n =18) and the mean response latency between BLSW.CAST-+/+ and BLSW.CAST-+/ ahl5 was not different. Together, these data indicate that the jams1 locus resides within the ahl5 critical interval. Gipc3 transgenic rescue To further test that the 343G>A mutation in Gipc3 causes the ahl5 and jams1 phenotypes, we generated transgenic animals expressing Gipc3 . Transgenic mice that were backcrossed to BLSW (N2–N3) were phenotyped using ABR at 6–8 weeks of age. In the control groups, Gipc3 343G/A heterozygotes, irrespective of the presence or absence of the transgene (tg(+/−)G/A), expressed normal hearing thresholds ( Fig. 3a and Supplementary Table S1 ) and Gipc3 343A/A homozygotes without the transgene (tg-A/A) exhibited the hearing loss characteristic of the ahl5 phenotype. Interestingly, Gipc3 343A/A homozygotes with the transgene (tg+A/A) showed hearing thresholds to the click, 8 and 16 kHz stimulus that were significantly lower than those of the tg-A/A mice. Furthermore, those thresholds were in the normal range and did not differ from those of the tg(+/−)G/A heterozygotes ( P >0.05). For the 32 kHz stimulus tg+A/A mice had thresholds that were elevated compared with tg(+/−)G/A heterozygotes (71±9 dBSPL; P <0.001), although these thresholds were still lower than those of tg-A/A (92±8 dBSPL). Next, transgenic and non-transgenic N2–N3 backcross mice were exposed to white noise at 3 weeks of age. Gipc3 343A/A homozygotes without the transgene (tg-A/A) reacted instantly at the 90 dBSPL stimulus with severe convulsions with an average latency period of 24 s. In contrast, Gipc3 343A/A homozygotes with the transgene (tg+A/A) showed a significant delay (108 s); none of the animals seized at the 90 dB stimulus and two animals showed a complete resistance ( Fig. 3b ). Gipc3 343G/A heterozygotes (tg(+/−)G/A) did not show any signs of seizing activity after 180 s of stimulation. In conclusion, the Gipc3 transgene rescued the ahl5 hearing deficit and jams1 audiogenic seizure susceptibility in Gipc3 343A/A homozygotes. 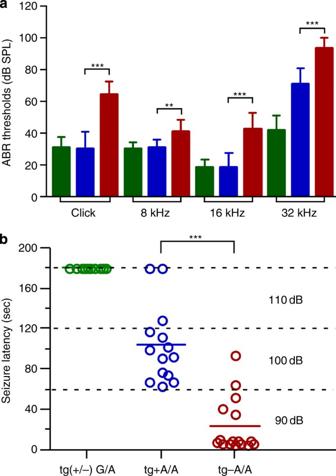Figure 3: Analysis of Gipc3 transgenic mice. (a) ABR thresholds (dBSPL) for click and pure tone pips at 8, 16 and 32 kHz are given in bars as mean±s.d. for backcross progeny tg(+/−) G/A (green,n=20), tg+A/A (blue,n=36) and tg-A/A (red,n=37). Green bars represent pooled data from backcross mice that were either positive or negative (+/−) for the transgene. (b) Audiogenic seizure susceptibility of tg(+/−) G/A (green symbol,n=10), tg+A/A (blue,n=) and tg-A/A (red,n=16) was assessed at 3 weeks of age using white noise stimuli (90, 100 and 110 dBSPL; dotted lines). Each circle represents one measurement and lines indicate the mean of the seizure latency of each genotype in seconds. **P<0.01; ***P<0.001. Figure 3: Analysis of Gipc3 transgenic mice. ( a ) ABR thresholds (dBSPL) for click and pure tone pips at 8, 16 and 32 kHz are given in bars as mean±s.d. for backcross progeny tg(+/−) G/A (green, n =20), tg+A/A (blue, n =36) and tg-A/A (red, n =37). Green bars represent pooled data from backcross mice that were either positive or negative (+/−) for the transgene. ( b ) Audiogenic seizure susceptibility of tg(+/−) G/A (green symbol, n =10), tg+A/A (blue, n =) and tg-A/A (red, n =16) was assessed at 3 weeks of age using white noise stimuli (90, 100 and 110 dBSPL; dotted lines). Each circle represents one measurement and lines indicate the mean of the seizure latency of each genotype in seconds. ** P <0.01; *** P <0.001. Full size image GIPC3 and human recessive deafness To test whether mutations in GIPC3 also underlie human SNHL, we screened panels of families of Dutch and Indian origin presenting with autosomal recessive nonsyndromic hearing impairment. In one Dutch family, W98-042, a homozygous region at 19p13.11-p13.3 encompassing GIPC3 was shared by the two affected siblings ( rs11880407 – rs6512152 ; assigned locus symbol: DFNB95). GIPC3 mutation analysis revealed a homozygous nucleotide substitution in exon 6, c.903G>A that segregated with the disease in the family ( Fig. 4a,b and Supplementary Table S2 ). The c.903G>A change is predicted to truncate the protein after residue 300 (p.Trp301X) causing the deletion of the C-terminal 12 amino acids of the protein. The mutation was not found in 156 (312 chromosomes) ethnically matched control individuals. 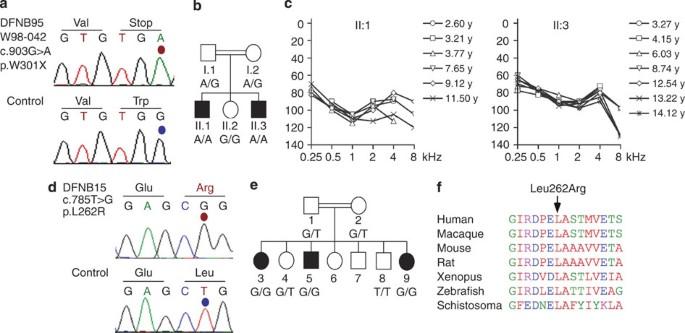Figure 4:GIPC3mutations and human deafness. (a) Sequencing chromatograms indicating the guanine (G) and adenine (A) in family W98-042 (top) and control (bottom) at nucleotide position c.903 changing the tryptophan (Trp) residue at position p.301 to a stop codon (p.Trp301X). (b) Shown is the two-generation pedigree of consanguinues family W98-042 with first-cousin parents. Hearing-impaired brothers homozygous for the mutation (II.I and II.3; A/A) are indicated by filled black boxes and normal hearing relatives are indicated by open symbols. (c) Mean pure-tone audiograms of the two affected individuals II.1 and II.3 of family W98-042 at different ages are given in years (y). Note the threshold shifts of 80–120 dB HL above normal hearing levels. (d) Sequence chromatogram showing c.785T>G (p.Leu262Arg) mutation inGIPC3in individual II-5. (e) Pedigree of the Indian family with prelingual, profound autosomal recessive non-syndromic hearing impairment. The c.785 genotype is shown. Open symbols unaffected; filled black symbols affected; double line consanguineous event. (f) Multi-sequence alignment of GIPC family proteins showing the high conservation of the Leu262 residue. Figure 4: GIPC3 mutations and human deafness. ( a ) Sequencing chromatograms indicating the guanine (G) and adenine (A) in family W98-042 (top) and control (bottom) at nucleotide position c.903 changing the tryptophan (Trp) residue at position p.301 to a stop codon (p.Trp301X). ( b ) Shown is the two-generation pedigree of consanguinues family W98-042 with first-cousin parents. Hearing-impaired brothers homozygous for the mutation (II.I and II.3; A/A) are indicated by filled black boxes and normal hearing relatives are indicated by open symbols. ( c ) Mean pure-tone audiograms of the two affected individuals II.1 and II.3 of family W98-042 at different ages are given in years (y). Note the threshold shifts of 80–120 dB HL above normal hearing levels. ( d ) Sequence chromatogram showing c.785T>G (p.Leu262Arg) mutation in GIPC3 in individual II-5. ( e ) Pedigree of the Indian family with prelingual, profound autosomal recessive non-syndromic hearing impairment. The c.785 genotype is shown. Open symbols unaffected; filled black symbols affected; double line consanguineous event. ( f ) Multi-sequence alignment of GIPC family proteins showing the high conservation of the Leu262 residue. Full size image The hearing loss in family W98-042 is bilateral and sensorineural with an early onset. Brainstem-evoked response audiometry for individual II.1 at 11 months of age revealed a threshold of ∼ 70 dB hearing levels (HL). For individual II.3 at the age of 3 months, brainstem-evoked response audiometry demonstrated a threshold of ∼ 80 dB HL. In individual II.1, the hearing loss progressed slowly to a loss of 110 dB at 12 years of age and individual II.3, who is now 14 years old, has a stable hearing loss of 90 dB HL ( Fig. 4c ). In an Indian family, segregating autosomal recessive non-syndromic hearing impairment previous linkage analyses detected a 32 cM region of homozygosity by descent at 19p13 ( D19S209 – D19S411; assigned locus symbol: DFNB15) that included the GIPC3 gene [24] . Sequencing of the six GIPC3 exons identified a homozygous missense mutation, c.785T>G (p.Leu262Arg), in exon 5 that segregated with the deafness in the family ( Fig. 4d,e and Supplementary Table S3 ). Sequence alignments of GIPC proteins indicated that the Leu262 residue is highly conserved ( Fig. 4f ). The mutation was not observed in 161 (322 chromosomes) control individuals. Hair bundle defects and sensorineural degeneration in BLSW The high-to-low frequency progression of the hearing loss suggested a histopathology in the organ of Corti. By confocal and scanning electron microscopy we observed an irregular structure of the stereocilia bundle of OHC and inner hair cells (IHC). Starting from postnatal day 3 (P3) onwards, OHC bundles were slightly disoriented and smaller, with bent lateral edges and a rounded apical pole ( Fig. 5a,b ). The hair bundle of IHC appeared less rigid and sparse ( Fig. 5a,b ) and at P21 stereocilia were thinner and at times also shorter ( Fig. 5c ). Stereocilia bundles at the base and mid-apical region were present and were affected to a similar degree. Histological sections of 8-week-old BLSW ears revealed a normal morphology of the organ of Corti and the spiral ganglion. At 52 weeks of age, there was a significant degeneration of the organ of Corti starting at the base and progressing towards the apex. Concomitantly, the spiral ganglion exhibited a severe loss of neurons that was most obvious at the base and the mid-apical region of the cochlea. The organ of Corti and spiral ganglion at the apex were of normal appearance ( Fig. 5d ). Together, these data suggest that Gipc3 is required for postnatal maturation of the hair bundle and long-term survival of hair cells and spiral ganglion. 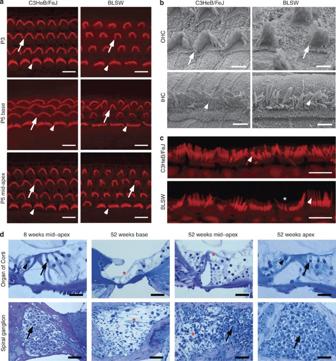Figure 5: Stereocilia and cochlear pathology in BLSW mice. (a) Confocal images of C3HeB/FeJ and BLSW phalloidin-stained organs of Corti at P3 and P5 from the mid-apical and basal turn are shown. Note the compromised hair bundle structure of OHC (white arrow) and collapsed bundle of IHC (arrowhead) in BLSW mice. Scale bar, 5 μm. (b) Shown are scanning electron microscopy images of OHC (arrow) and IHC (arrowhead) stereocilia bundles at P14. Compare the inward-bended stereocilia on BLSW OHCs to the organized and upright standing bundles in C3HeB/FeJ. Compare the sparse IHC stereocilia in BLSW with the dense bundle in C3HeB/FeJ. Scale bar, 2 μm. (c) Shown are confocal images of IHC stereocilia bundles at P21. Note the thinner (arrow) and shorter (star) stereocilia in BLSW. Scale bar, 5 μm. (d) Images of tolouidine-stained cross-sections of the organ of Corti and spiral ganglion are shown. Age and region of the cochlea is indicated. Note the normal appearance of organ of Corti (arrows point to OHC and arrowhead to IHC) and spiral ganglion neurons (arrow) in 8-week-old BLSW mice, but base to mid–apex degeneration (red star) in 52-week-old BLSW cochleae. Scale bar, 20 μm (top panel) and 50 μm (bottom panel). Figure 5: Stereocilia and cochlear pathology in BLSW mice. ( a ) Confocal images of C3HeB/FeJ and BLSW phalloidin-stained organs of Corti at P3 and P5 from the mid-apical and basal turn are shown. Note the compromised hair bundle structure of OHC (white arrow) and collapsed bundle of IHC (arrowhead) in BLSW mice. Scale bar, 5 μm. ( b ) Shown are scanning electron microscopy images of OHC (arrow) and IHC (arrowhead) stereocilia bundles at P14. Compare the inward-bended stereocilia on BLSW OHCs to the organized and upright standing bundles in C3HeB/FeJ. Compare the sparse IHC stereocilia in BLSW with the dense bundle in C3HeB/FeJ. Scale bar, 2 μm. ( c ) Shown are confocal images of IHC stereocilia bundles at P21. Note the thinner (arrow) and shorter (star) stereocilia in BLSW. Scale bar, 5 μm. ( d ) Images of tolouidine-stained cross-sections of the organ of Corti and spiral ganglion are shown. Age and region of the cochlea is indicated. Note the normal appearance of organ of Corti (arrows point to OHC and arrowhead to IHC) and spiral ganglion neurons (arrow) in 8-week-old BLSW mice, but base to mid–apex degeneration (red star) in 52-week-old BLSW cochleae. Scale bar, 20 μm (top panel) and 50 μm (bottom panel). Full size image Reduced Gipc3 protein levels in the BLSW cochlea We reasoned that the Gly115Arg mutation might alter the expression or stability of Gipc3. To test this hypothesis, we probed western blots with polyclonal antisera raised against Gipc3-specific peptides. In protein extracts derived from HEK293T cells transiently expressing wild-type Gipc3 , the Pb867, Pb869 and Pb877 antisera detected a single ∼ 40 kDa immunoreactive band ( Fig. 6a and Supplementary Fig. S2 ). When we probed western blots of cochlea and testis protein extracts from BLSW and C3HeB/FeJ we detected a reduction in intensity of the ∼ 40 kDa band in BLSW cochlea extracts by 82±7% ( n =3) and in testis extracts by 42±9% ( n =3) compared with wild-type C3HeB/FeJ extracts ( Fig. 6b ). As an additional test of the expression level differences, we generated a mutant Gipc3 343A cDNA construct for expression in HEK293T cells. Quantification, after normalizing against actin expression, revealed a reduction in expression levels by 69% of the mutant Gipc3(115Arg) protein compared with that for wild-type Gipc3(115Gly) ( Fig. 6c,d ). TaqMan qPCR analyses revealed no significant differences in Gipc3 mRNA expression in HEK293T cells transfected with wild-type ( Gipc3 343G ) or mutant ( Gipc3 343A ) construct (data not shown). In addition to the ∼ 40 kDa band, Pb867 recognizes a ∼ 37 kDa band in both cochlea and testis extracts. Both bands can be blocked by the Gipc3-specific peptide used for generating the Pb867 antibody and are also detected by the Pb869/Pb877 antiserum ( Supplementary Fig. S2 ). In addition, Pb867 is specific for Gipc3, showing strong reactivity with human GIPC3 and only faint cross reactivity with mouse Gipc1 and Gipc2 ( Supplementary Fig. S2 ). Thus, the ∼ 37 kDa band may represent either an alternate isoform or partially cleaved product of the ∼ 40 kDa protein. Together, these data indicate that the Gly115Arg substitution causes a reduction of the 40 kDa Gipc3 protein in BLSW cochleae. 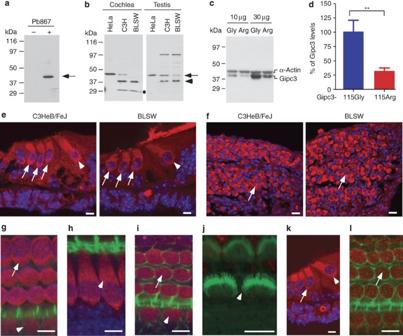Figure 6: Protein blot analysis and immunolocalization of Gipc3. (a) Western blot analysis ofGipc3343Gtransfected (+) and untransfected (−) HEK293T cell lysates using Gipc3-specific polyclonal antiserum Pb867 detecting a single∼40 kDa band (black arrow). (b) Immunoblot analysis of protein extracts from cochlea and testis from BLSW and C3HeB/FeJ (C3 H) mice with anti-Gipc3 antiserum Pb867. Lysates from HeLa cells transfected with the wild-typeGipc3343Gconstruct were included as control. The∼40 kDa band (black arrow) was detected in both tissues from C3HeB/FeJ wild-type mice. The similar∼40 kDa band was detected with reduced intensity in mutant BLSW cochlea and testis. The∼37 kDa band (arrow head) and∼29 kDa band (dot, presumably nonspecific) are indicated. (c) Quantitative analysis of wild-type Gipc3(115Gly) and mutant Gipc3(115Arg) expression in lysates from transiently transfected HEK293T cells with varying amounts of protein loaded (10 and 30 μg) for wild-typeGipc3343Gand mutantGipc3343A. Protein blots were probed with the anti-Gipc3 antiserum Pb867and anti-α-actin antibody. (d) Densitometric analysis of Gipc3 expression from wild-type Gipc3(115Gly) and mutant Gipc3(115Arg)-transfected HEK293T cells. The data are represented as mean±s.e.m., **P<0.01 (n=6,t-test). Confocal images of cryosections of organ of Corti (e) and spiral ganglion (f) stained with Pb867 antibody (red) demonstrating Gipc3 localization in IHCs (arrow head) and OHCs (arrow) and spiral ganglion (arrow). Confocal images of organ of Corti of C3HeB/FeJ (g,h,j) and BLSW (i,k,l) demonstrating Gipc3 (g–i) and Vglut3 (k) and myosin VI (l) localization; (i–l) counterstained with phalloidin (green); arrows point to positive staining. (e–k) Counterstained with 4,6-diamidino-2-phenylindole (blue). (l) No Pb867-staining is seen in stereocilia of IHC (arrow head); scale bar, 5 μm (e–l). Figure 6: Protein blot analysis and immunolocalization of Gipc3. ( a ) Western blot analysis of Gipc3 343G transfected (+) and untransfected (−) HEK293T cell lysates using Gipc3-specific polyclonal antiserum Pb867 detecting a single ∼ 40 kDa band (black arrow). ( b ) Immunoblot analysis of protein extracts from cochlea and testis from BLSW and C3HeB/FeJ (C3 H) mice with anti-Gipc3 antiserum Pb867. Lysates from HeLa cells transfected with the wild-type Gipc3 343G construct were included as control. The ∼ 40 kDa band (black arrow) was detected in both tissues from C3HeB/FeJ wild-type mice. The similar ∼ 40 kDa band was detected with reduced intensity in mutant BLSW cochlea and testis. The ∼ 37 kDa band (arrow head) and ∼ 29 kDa band (dot, presumably nonspecific) are indicated. ( c ) Quantitative analysis of wild-type Gipc3(115Gly) and mutant Gipc3(115Arg) expression in lysates from transiently transfected HEK293T cells with varying amounts of protein loaded (10 and 30 μg) for wild-type Gipc3 343G and mutant Gipc3 343A . Protein blots were probed with the anti-Gipc3 antiserum Pb867and anti-α-actin antibody. ( d ) Densitometric analysis of Gipc3 expression from wild-type Gipc3(115Gly) and mutant Gipc3(115Arg)-transfected HEK293T cells. The data are represented as mean±s.e.m., ** P <0.01 ( n =6, t -test). Confocal images of cryosections of organ of Corti ( e ) and spiral ganglion ( f ) stained with Pb867 antibody (red) demonstrating Gipc3 localization in IHCs (arrow head) and OHCs (arrow) and spiral ganglion (arrow). Confocal images of organ of Corti of C3HeB/FeJ ( g , h , j ) and BLSW ( i , k , l ) demonstrating Gipc3 ( g–i ) and Vglut3 ( k ) and myosin VI ( l ) localization; ( i – l ) counterstained with phalloidin (green); arrows point to positive staining. ( e – k ) Counterstained with 4,6-diamidino-2-phenylindole (blue). ( l ) No Pb867-staining is seen in stereocilia of IHC (arrow head); scale bar, 5 μm ( e – l ). Full size image Gipc3 localization in hair cells and ganglion neurons Using the Pb867 antibody on cochlear sections, we detected Gipc3-specific immunoreactivity in IHCs and OHCs, as well as in cochlear spiral ganglion neurons in C3HeB/FeJ mice. Similar expression domains were observed in the BLSW cochlea ( Fig. 6e,f ). Staining was also present in the cytoplasm of vestibular hair cells and vestibular ganglion neurons ( Supplementary Fig. S2 ). On whole-mount organ of Corti preparations, we noted abundant staining in the cytoplasm of IHCs and OHCs characterized by fine punctate staining apparent at the base, around the nucleus and throughout the apical part of the hair cells ( Fig. 6g–i ). There was no obvious staining at the stereocilia bundle ( Fig. 6j ). Immunostaining with Pb877 revealed a similar expression and localization profile, showing staining of the cytoplasm of vestibular and cochlear hair cells and spiral ganglion neurons ( Supplementary Fig. S2 ). Staining with antibodies against Vglut3 and Myosin VI showed localizations similar with Gipc3 in BLSW cochleae ( Fig. 6k,l ). Incubation with nonspecific rabbit IgG antiserum produced no staining ( Supplementary Fig. S2 ). Mechanotransduction and K + currents in BLSW The compromised structure of the stereocilia bundle suggested a defect in mechanotransduction. At P6, we found no difference in transduction currents recorded from OHCs and IHCs between BLSW and Swiss Webster control mice. The mean maximal amplitudes of the transduction currents operating range and adaptation time constants were not significantly different between BLSW and control hair cells. However, by P12 we observed a significant reduction in the maximal transduction current amplitude in both IHCs and OHCs. The mean maximal transduction currents recorded from IHCs and OHCs of P12-P14 BLSW mice were reduced by 57 and 71%, respectively, compared with control hair cells ( Fig. 7a,b ). This reduction likely accounts for the elevated hearing thresholds. 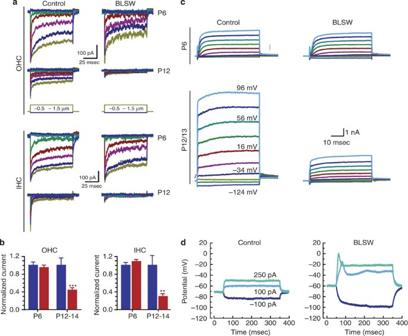Figure 7: Electrophysiological measurements from BLSW and control mice. (a) Families of transduction currents recorded from OHC (n=8–11) and IHC (n=3–10) collected from the apical turn of BLSW and control mice at P6 and P12 are shown. The scale bar applies to all four families. The cells were voltage-clamped at −64 mV. The data shown at P6 are representative of the mean, whereas the data shown at P12 represent the largest currents obtained at that stage. (b) Summary of mean maximal currents recorded from a total of 62 hair cells of control (blue bars) and BLSW (red). The data were normalized to mean maximal control currents in each condition. Bars indicate mean±s.e.m.; **P<0.005; ***P<0.00005 (two-populationt-test). (c) Families of voltage-dependent currents evoked by 50-msec steps that ranged between −124 and 96 mV in 20 mV increments. Currents were recorded from IHC at P6 (top panel) and at P13 (control,n=5) and P12 (BLSW,n=8, bottom panel). The scale bar applies to all current families. (d) Membrane potentials recorded in current-clamp mode in response to current steps at the amplitudes indicated. Figure 7: Electrophysiological measurements from BLSW and control mice. ( a ) Families of transduction currents recorded from OHC ( n =8–11) and IHC ( n =3–10) collected from the apical turn of BLSW and control mice at P6 and P12 are shown. The scale bar applies to all four families. The cells were voltage-clamped at −64 mV. The data shown at P6 are representative of the mean, whereas the data shown at P12 represent the largest currents obtained at that stage. ( b ) Summary of mean maximal currents recorded from a total of 62 hair cells of control (blue bars) and BLSW (red). The data were normalized to mean maximal control currents in each condition. Bars indicate mean±s.e.m. ; ** P <0.005; *** P <0.00005 (two-population t -test). ( c ) Families of voltage-dependent currents evoked by 50-msec steps that ranged between −124 and 96 mV in 20 mV increments. Currents were recorded from IHC at P6 (top panel) and at P13 (control, n =5) and P12 (BLSW, n =8, bottom panel). The scale bar applies to all current families. ( d ) Membrane potentials recorded in current-clamp mode in response to current steps at the amplitudes indicated. Full size image To examine voltage-dependent channel activity, we delivered 50-msec voltage steps and measured families of potassium currents from IHCs. At P6, both control and BLSW IHCs had currents with similar amplitudes and kinetics. By P13, control cells had acquired a large rapidly activating potassium current (1726±323 pA at 0 mV) consistent with previous reports [25] . In contrast, potassium currents from IHC of BLSW mice at P12 had significantly smaller amplitudes (869±323 pA at 0 mV; P <0.01; t -test) not unlike those at P6, albeit with faster activation kinetics ( Fig. 7c ). To consider the functional impact of the attenuated current amplitudes in the BLSW IHCs, we switched to current-clamp mode and delivered current steps of −100, 100 and 250 pA. Control cells had small membrane potentials consistent with a previous report on wild-type responses [25] , but in BLSW mice the responses were substantially larger, with depolarizations that reached well into the range of calcium channel activation (positive to –60 mV; Fig. 7d ). ABR amplitudes and audiogenic seizure progression To investigate the cause of the audiogenic seizure susceptibility and resistance, we correlated various ABR output parameters with seizure progression. Acoustic stimulation showed that BLSW mice were most susceptible to seizures between 2 and 4 weeks of age with mean seizure latencies of 40±42 s ( n =19) and 89±32 s ( n =21), respectively. Thereafter, latencies increased until animals became completely resistant at 6 weeks of age (180 s, n =15). Increases in seizure latencies were significant between 3 and 5 weeks and between 4 and 6 weeks of age ( Fig. 8a ). 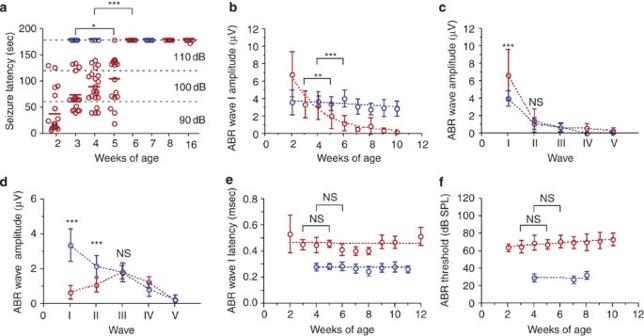Figure 8: Audiogenic seizure progression correlates with ABR wave I amplitude. (a) Shown are audiogenic seizure latencies (seconds) after white noise stimulation at 90, 100 and 110 dBSPL (dotted lines) of BLSW (red,n≥9) and C3HeB/FeJ (blue,n≥3) as function of weeks of age. Each circle represents one measurement and the line indicates the mean of the response. (b) Shown are ABR wave I amplitudes obtained with a 100-dBSPL click stimulus of BLSW (red,n≥8) and C3HeB/FeJ (blue,n≥9) as function of weeks of age. Data are given as mean±s.d. (c,d) Shown are ABR amplitudes for waves I through V following a 100-dBSPL click stimulus of BLSW (red,n≥9) and C3HeB/FeJ (blue,n≥10) at 2 (c) and 6 (d) weeks of age. Data are given as mean±s.d. (e) Shown are ABR wave I latencies obtained with a 100-dBSPL click stimulus of BLSW (red,n≥8) and C3HeB/FeJ (blue,n≥9) as function of weeks of age. Data are given as mean±s.d. (f) ABR thresholds shown are obtained with a click stimulus of BLSW (red,n≥9) and C3HeB/FeJ (blue,n≥2) as function of weeks of age. Data are given as mean±s.d. Dotted connecting lines: linear regression lines. NSP>0.05; *P<0.05; **P<0.01; ***P<0.001, ANOVA. NS, not significant. Figure 8: Audiogenic seizure progression correlates with ABR wave I amplitude. ( a ) Shown are audiogenic seizure latencies (seconds) after white noise stimulation at 90, 100 and 110 dBSPL (dotted lines) of BLSW (red, n ≥9) and C3HeB/FeJ (blue, n ≥3) as function of weeks of age. Each circle represents one measurement and the line indicates the mean of the response. ( b ) Shown are ABR wave I amplitudes obtained with a 100-dBSPL click stimulus of BLSW (red, n ≥8) and C3HeB/FeJ (blue, n ≥9) as function of weeks of age. Data are given as mean±s.d. ( c , d ) Shown are ABR amplitudes for waves I through V following a 100-dBSPL click stimulus of BLSW (red, n ≥9) and C3HeB/FeJ (blue, n ≥10) at 2 ( c ) and 6 ( d ) weeks of age. Data are given as mean±s.d. ( e ) Shown are ABR wave I latencies obtained with a 100-dBSPL click stimulus of BLSW (red, n ≥8) and C3HeB/FeJ (blue, n ≥9) as function of weeks of age. Data are given as mean±s.d. ( f ) ABR thresholds shown are obtained with a click stimulus of BLSW (red, n ≥9) and C3HeB/FeJ (blue, n ≥2) as function of weeks of age. Data are given as mean±s.d. Dotted connecting lines: linear regression lines. NS P >0.05; * P <0.05; ** P <0.01; *** P <0.001, ANOVA. NS, not significant. Full size image Amplitudes of the first (I) ABR wave (click at 100 dBSPL) were significantly higher in 2-week-old BLSW mice (6.8±2.6 μV, n =24) compared with control C3HeB/FeJ mice (3.9±1.0 μV, n =12). These high amplitudes declined rapidly to 0.55±0.25 μV ( n =10) at 7 weeks of age. In particular, decreases in wave I amplitudes were significant between 3 (3.5±1.5 μV, n =18) and 5 (2.1±1.5 μV, n =24) and between 4 (3.3±1.5 μV, n =33) and 6 (1.2±0.9 μV, n =32) weeks of age ( Fig. 8b ). In contrast, the wave I amplitude in control mice remained constant over the 8-week test period, showing no difference between 2- and 10-week-old mice (2.9±0.8 μV, n =10, P >0.05). Amplitudes of waves II through V were not significantly different between BLSW and controls at 2 weeks of age. At 6 weeks of age the amplitude of wave II was reduced in BLSW, but the amplitudes of waves III through V were not diffierent compared with C3HeB/FeJ control ( Fig. 8c,d ). We next analysed the latency of the ABR wave I. Latencies of 3- to 10-week-old BLSW mice were on average 0.14 ms higher than those in control mice ( P <0.001), but did not change significantly over the test period ( P >0.05). Specifically, no significant delays were observed between 3 (0.4±0.04 ms, n =10) and 5 (0.4±0.03, n =8) and between 4 (0.4±0.05 ms, n =9) and 6 (0.4±0.04, n =17) weeks of age ( Fig. 8e ). Last, we correlated ABR thresholds at the click stimulus with seizure progression. ABR thresholds slightly increased in BLSW mice between 2 and 12 weeks of age. However, there were no significant increases in thresholds in mice between 3 (65±6 dBSPL, n =33) and 5 (67±6 dBSPL, n =27) and between 4 (69±8 dBSPL, n =32) and 6 weeks of age (71±7 dBSPL, n =24; Fig. 8f ). Together, these data suggest that the elevated and subsequent decline of the wave I amplitude correlated with the susceptibility and resistance to audiogenic seizures, respectively. Despite significant advances in the understanding of monogenic deafness, the molecular genetics of the more common and complex forms of hearing loss is poorly characterized. Nine QTLs controlling oligogenic hearing impairment in the mouse have been reported, but, thus far, only two loci have been molecularly characterized ( Cdh23 753A and Fscn2 326A ) [26] , [27] . Here, we identified the ahl5 / jams1 and DFNB15/DFNB95 loci uncovering a function for Gipc3 in peripheral auditory signal transmission in mouse and human. Gipc3 distribution in hair cells is reminiscent of vesicular staining and shows a similar localization as Vglut3 and Myosin VI, proteins that regulate synaptic glutamate release and Ca 2+ -dependent exocytosis at the IHC ribbon synapse, respectively [28] , [29] , [30] . GIPC1 was shown to associate with membranous and cytosolic fractions and also localizes to synaptic vesicles at presynaptic axon terminals of hippocampal neurons [19] , [31] . Interestingly, glutamate release from presynaptic terminals in the hippocampus was shown to depend on GIPC1/Myo6 interactions [19] . Given the hair bundle defect, reduced mechanotransduction and K + currents as well as abnormal ABR wave I amplitude in BLSW mice, we hypothesize that Gipc3 may be part of a protein complex involved in vesicle trafficking that transports factors critical for signal aquisition and propagation in cochlear hair cells. The Gly115Arg change occurring in the loop connecting the βB with the βC strand of the PDZ domain is positioned closely to the peptide recognition pocket [32] . Our western blot data indicate that the Gly115Arg substitution leads to a reduction in Gipc3 protein levels. It is possible that a conformational change or loss of stable interactions may target Gipc3(115Arg) for early degradation. The human Trp301X mutation truncates a peptide that shows 42% sequence identity with the GIPC1 C-terminus. It was recently shown that truncation of 29 residues of the C-terminus of GIPC1 abolishes interaction with Myosin VI suggesting that the full-length C-terminus is required to form stable interactions [33] . In addition, both Leu262 and Trp301 residues are highly conserved among metazoan GIPC proteins. These data indicate that Trp301X and Leu262Arg are pathogenic mutations. It was recently suggested that the transient audiogenic seizures in BLSW mice occur independent of the hearing loss [12] . Indeed, our data do not support a correlation between hearing thresholds and audiogenic seizure progression. Furthermore, the reduced mechanosensitivity seems to be at odds with audiogenic seizure susceptibility. However, our results implicate the ABR wave I amplitude, which represents the summed activity of the cochlear nerve fibres projecting from IHCs to the cochlear nucleus, in seizure susceptibility and resistance [34] . The high wave I amplitude at 2 weeks of age may result from the stunted developmental acquisition of IHC K + currents. Whereas the normal acquisition of potassium currents attenuates the IHC receptor potential, lack of those currents in BLSW allows greater depolarization, which may in turn enhance Ca 2+ -dependent neurotransmission, perhaps leading to synchronized cochlear nerve activity, enhanced ABR wave I amplitudes and seizure susceptibility. The subsequent decline in the ABR wave I amplitude and seizure resistance in BLSW mice may be indicative of a neuropathy at the IHC spiral ganglion neuron synapse. In the cochlea, glutamate receptors mediate fast synaptic transmission at the IHC afferent synapse and glutamate excitotoxicity is central to the neural damage during acoustic trauma [35] , [36] . Clinically, the audiogenic seizure pathology in BLSW mice is a form of reflex epilepsy, in which external sensory stimuli induce seizures. In humans, acoustic reflex epilepsies, although rare, include startle and musicogenic epilepsies and overt sensitivity to sound also underlies hyperacusis and hyperacute hearing in autism syndrome [37] , [38] , [39] , [40] . The pathogeneses underlying these sensitivities are not understood or is it clear whether they originate in the central or peripheral auditory system. BLSW mice and perhaps other mutant alleles of Gipc3 may prove critical to better understand the cause of acoustic hypersensitivity. Our analysis of the hearing loss in BLSW mice has interesting implications for the genetics of human progressive SNHL. GIPC3 and its paralogs are excellent candidate genes for ARHI. It can be argued that ahl5 is a monogenic trait not modelling the degree of genetic complexity presumed to underlie AHRI. Although this argument assumes the common variant-common disease hypothesis, it is also conceivable that rare alleles with strong effects in homozygous or heterozygous state may be strong contributors to ARHI. Furthermore, a mutation in the grainyhead like 2 gene ( GRHL2 ) causes progressive hearing loss in humans and a candidate gene approach subsequently associated a GRHL2 variant with ARHI [41] , [42] . Susceptibility to metabotropic glutamate receptor 7 (mGluR7)-mediated excitotoxicity was suggested as risk factor for ARHI [3] . Interestingly, mGluR7 and Gipc3 show identical localization domains in the mouse cochlea and also share functional similarities [3] , [18] . Primary neuronal degeneration, which causes hearing impairment because of spiral ganglion degeneration in the absence of hair cell loss, was recently shown to underlie the long-term effect of noise exposure [43] . Likewise, hearing loss in BLSW mice at 8 weeks of age occurs without a noticeable hair cell loss. Together, these observations suggest a prominent role for variations in genes affecting spiral ganglion function in sensorineural progressive hearing loss. Mice and crosses Black Swiss mice were obtained from Taconic and C3HeB/FeJ mice were purchased from The Jackson Laboratory. BLSW mice were originally generated by outcrossing albino NIH Swiss mice to C57BL/6N and then backcrossing to the NIH Swiss line selecting for black coat colour [44] . In our colony, BLSW mice are maintained by brother × sister mating. To generate BLSW × CAST/EiJ congenic lines (here referred to as BLSW.CAST- +/ahl5 ), N2 backcross mice [11] that were heterozygous over a 25 Mbp region on chromosome 10 and showed normal hearing thresholds were serially backcrossed to BLSW. At each generation, we assessed the hearing phenotype at 8 weeks of age using ABR threshold measurements at four stimuli (click, 8, 16 and 32 kHz) and genotyped markers located every 10cM along chromosome 10 and markers within the D10Mit20 and D10Mit95 interval. To generate Gipc3 transgenic mice, a 3292 kbp PaqI DNA fragment of the pBROAD-Gipc3 clone containing the mouse ROSA26 promoter, Gipc3 coding sequence and human β-globin polyadenylation sequence was injected into FVB/N-derived male pronuclei. Transgenic animals were serially backcrossed to BLSW and genotyped by PCR. Institutional review boards at NIH and University of Virginia approved the animal studies. Auditory tests in mice For ABR, acoustic stimuli were generated from a high frequency transducer and presented at varying intensity at a rate of 19.1 times per s for a total of 350 presentations. Neuronal responses were captured through subdermal needle electrodes inserted at the vertex, filtered, amplified and displayed. Thresholds, latencies and amplitudes were determined using IHS software. DPOAEs were measured using National Instruments (NI) LabView 8.6 software, operating an NI PCI-4461 Dynamic Signal Analyzer sound card (National Instruments), to generate two pure tones, f1 and f2, at the fixed f2/f1 ratio of 1.25, which were emitted separately by two Clarion SRU310H high frequency dome tweeters (Clarion) placed in the outer ear canal at the presentation level of f2=f1. Emissions were measured using an Etymõtic-ER-10B+ microphone. The amplitude of the 2f1-f2 distortion product was plotted in dBSPL against the f2 frequency where the distortion product is generated. To measure the EP, a silver/chloride electrode bathed in 0.1 M KCl was inserted through the round window into the endolymph using a remote controlled motorized Micromanipulator (Piezo World Precision Instrument). The electrode was connected to a Warner Dual Channel Differential Electrometer (HiZ-223; Warner Instruments), which amplified and routed the voltage difference (subdermal 1 M KCl reference electrode) to the data acquisition system (Digidata 1440A, Axon Instruments) using AxoScope software (Axon) at a sampling rate of 10 kHz for 60 s. To induce audiogenic seizures, mice were exposed to white noise of 90, 100 and 110 dBSPL consecutively for 60 s each stimulus. Acoustic stimuli were generated by a Bose loudspeaker (Bose) operated by ToneGen software. Speaker levels were calibrated with SoundProDL (Clarke Analytical Instruments). The mouse was placed in a clear polypropylene box container with a lid with the loud speaker mounted into the side. Each stimulus was maintained for 60 s or until a seizure occurred as evidenced by wild running, flexing and tonic-clonic convulsions [45] . Seizure latency (sec) was defined as the time of the first stimulus onset to the time of seizure onset. Animals resistant to the three consecutive sound stimuli were scored as having a latency of 180 s. To measure mechanotransduction, the hair bundles were stimulated with a fire polished glass probe that fit the shape of the bundles. The stimulator was cemented to a PICMA ultra fast piezo actuator (Physik Instrumente), driven by a ENV-400 amplifier (Piezosystem Jena). Transduction currents were recorded using the whole-cell, tight-seal technique. Recording pipettes were filled with intracellular solution. Membrane potential was clamped to −64 mV and controlled using an Axopatch Multiclamp 700A amplifier (Molecular Devices). pClamp 8.2 (Molecular Device) and Origin 7.5 (OriginLab) were used to record and analyse the currents. Antibodies and immunoblot analysis Rabbit polyclonal antisera (Covance) were raised against Gipc3-specific peptides (Princeton Biomolecules). Sera were affinity-purified (Covance). Antiserum Pb867 was raised against EPPARARPRLVFRTQLAHGS (aa 13–32); Pb869: APSDVEAAAARRVDDL (aa 220–235); Pb877 VSSGRETLRLRSGGAATVEEA (aa 199–220). Mouse Gipc3 protein reference sequence: NP_683753, GenBank protein sequence database. Additional antibodies used are Anti-Myosin VI (Sigma) and Anti-Vglut3 (SynapticSystem). Cochleae and testis were homogenized in RIPA buffer containing 1 mM phenylmethylsulphonyl fluoride and complete protease inhibitor cocktail (Roche). Confluent HEK293 or HeLa cells were lysed on ice in 20 mM Tris-HCl (pH 6.8), 150 mM NaCl, 10 mM EDTA, 1 mM EGTA, 10 mM iodoacetamide, 1% Triton X-100 with complete protease inhibitor cocktail (Roche). For immunoblots, the protein lysate was resolved by 4–12% SDS polyacrylamide gel electrophoresis, transferred to nitrocellulose membrane, incubated with the primary antibody, complexed with a secondary goat anti-rabbit or goat anti-mouse antibody conjugated to horseradish peroxidase (Kirkegaard and Perry Laboratories) and detected using enhanced Chemiluminescence (Pierce Laboratories). The data were quantified by measuring total protein band intensities ratios using UVP multispectral imaging system and normalized to control α-actin band. Histology and immunohistochemistry For gross morphology, the ear was fixed with 4% paraformaldehyde, decalcified, dehydrated with a graded series of ethanol, and infiltrated with JB-4 polymer. Serial sections were cut at 4 μm thickness and stained with 0.1% Toluidine Blue O. For cryosections, ears were fixed, equilibrated in a graded series of sucrose in PBS, transferred to a 2:1 mixture of 20% Sucrose in PBS:OCT Medium (Saukra), frozen over dry ice and ethanol, and sectioned at 12 μm. For immunostaining of whole-mounts of organ of Corti, cochlea ducts were dissected in Leibovitz and fixed. Specimens were permeabilized in 0.5% TritonX-100, incubated with affinity-purified antibody Pb867 (1:1000) and secondary anti-rabbit IgG (1:1000; Alexa Fluor 594). For visualizing the stereociliary bundle, the specimen was stained with Rhodamine phalloidin (Invitrogen) diluted 1:100 in PBS, mounted in ProLong Gold antifade and imaged using a Zeiss LSM confocal microscope. For scanning electron microscopy, ears were fixed in 4% glutaraldehyde, 3 mM CaCl 2 , 0.1M HEPES pH 7.4, dissected, washed in PBS, post-fixed in 1% OsO 4 , dehydrated in ethanol, critical point dried, sputter coated with platinum and imaged in a Field emission scanning electron microscope (Hitachi, S-4500). Plasmid constructs and transfections Full-length mouse Gipc3 (ref. sequence: NM_148951 , GenBank Nucleotide Core) was amplified from CBA/CaJ cochlea cDNA by PCR and cloned into pCR4-TOPO vector (Invitrogen) to generate clone pU2. For the transgene construct, a 932-bp Eco RI restriction fragment from plasmid pU2 was cloned into pBROAD3-mcs vector (InvivoGen) to generate clone pBroad-Gipc3. For transfection experiments, the 932-bp wild-type cDNA Gipc3 from clone pU2 was cloned in pcDNA3.1(+) as a Eco RI fragment to create clone pcDNA3.1- Gipc3 . Mutant pcDNA3.1- Gipc3 343A was generated by site-directed mutagenesis using QuickChange mutagenesis kit (Stratagene). Constructs were verified by DNA sequencing using the BigDye Terminator v 3.1 following the manufacturer's instructions and electrophoresed on a 3730xl capillary sequencer (Applied Biosystems). For transient expression, Lipofectamine (Invitrogen) was used to transfect HEK293T or HeLa cells with a constant amount of plasmid DNA (1 μg or 2 μg) of pcDNA3.1- Gipc3 or pcDNA3.1- Gipc3 343A . Total protein extraction for western blot was performed 48 h after transfection. Molecular genetic analyses in mice To sequence coding exons in the ahl5 interval, genomic sequences were obtained from http://genome.ucsc.edu and PCR primers flanking the exons were designed using Primer3 http://Frodo.wi.mit.edu . Exons were amplified and cycle sequencing was performed as described above. Sequence chromatograms were analysed using Sequencher v4.5 (Gene Code Corporation). BLSW DNA sequences were compared against the C57BL/6J reference sequence. Presence of the Gipc3 343G > A mutation was evaluated by DNA sequencing. Human patients and mutation analysis The local medical ethics committees at the Radboud University Nijmegen, the Netherlands, the University of Iowa, USA and the University of Madras, India approved the studies. Informed consent was obtained from the participating subject or, in the case of children, from their parents. For the DFNB95 family, members were examined by otoscopy and pure-tone audiometry in a sound-treated room in accordance with current clinical standards. Individual II.1 received a cochlear implant after the audiogram taken at 11.5 years of age. High-resolution single-nucleotide polymorphism (SNP) genotyping and mutation analysis was performed as described [46] . Briefly, genome-wide linkage scans were performed using the Affymetrix mapping 250K SNP array (Affymetrix). Genotypes and regions of homozygosity were defined using the Genotyping Console software (Affymetrix). Primers for amplification of exons and exon–intron boundaries of GIPC3 were designed with ExonPrimer according to the reference sequences NM_133261.2 and NT_011255.14 ( Supplementary Table S2 ). To determine the segregation of the c.903G>A variant in the family and the presence in normal controls, exon 6 was amplified and the PCR product was digested with Sau96I (New England Biolabs). The DFNB15 locus segregating in a two-generation consanguineous Indian family with prelingual, profound autosomal recessive hearing impairment was reported previously [24] . The GIPC3 gene was amplified using gene-specific primers using a standard protocol on a GeneMate Genius thermocycler (ISC BioExpress), sequenced and analysed as described above. Statistical analyses Unless otherwise indicated groups of data were compared using one-way ANOVA followed by Bonferroni post-tests to correct for multiple testing. GraphPad Prism 4.0b software (GraphPad) was used to perform the arithmetic, statistics and to plot the data. Accession Code: The mouse GIPC3 sequence ( NM_148951 , GenBank Nucleotide Core) and protein ( NP_683753 , GenBank protein sequence database) accession codes were used in this study. How to cite this article: Charizopoulou, N. et al . Gipc3 mutations associated with audiogenic seizures and sensorineural hearing loss in mouse and human. Nat. Commun. 2:201 doi: 10.1038/ncomms1200 (2011).